Individual diet has sex-dependent effects on vertebrate gut microbiota Vertebrates harbour diverse communities of symbiotic gut microbes. Host diet is known to alter microbiota composition, implying that dietary treatments might alleviate diseases arising from altered microbial composition (‘dysbiosis’). However, it remains unclear whether diet effects are general or depend on host genotype. Here we show that gut microbiota composition depends on interactions between host diet and sex within populations of wild and laboratory fish, laboratory mice and humans. Within each of two natural fish populations (threespine stickleback and Eurasian perch), among-individual diet variation is correlated with individual differences in gut microbiota. However, these diet–microbiota associations are sex dependent. We document similar sex-specific diet–microbiota correlations in humans. Experimental diet manipulations in laboratory stickleback and mice confirmed that diet affects microbiota differently in males versus females. The prevalence of such genotype by environment (sex by diet) interactions implies that therapies to treat dysbiosis might have sex-specific effects. Animals live in intimate association with diverse communities of symbiotic bacteria [1] , [2] . Intestinal microbial communities are particularly abundant and diverse, and promote host development, nutrition and immunity [3] , [4] , [5] , [6] . When the microbiota is perturbed (‘dysbiosis’), these services may be disrupted, leading to disorders including obesity, diabetes and inflammation [5] , [7] , [8] , [9] . Consequently, there is growing interest in the possibility of manipulating the microbiota to treat diseases arising from dysbiosis. Such therapeutic interventions require a detailed understanding of the ecological, genetic and physiological processes that structure symbiotic microbial communities. Microbial taxon composition and relative abundance varies dramatically among host individuals even within a single host population. This among-host variation provides an opportunity to study processes that structure the microbiota. It is now clear, for example, that microbiota composition depends on both individual genotype [10] , [11] , [12] and environment [13] , [14] , [15] , [16] . Environmental factors such as diet [15] , [17] are of particular interest as a cost-effective means for therapeutic alteration of gut microbiota [18] , [19] . Unfortunately, most studies of gut microbiota regulation evaluate host genetic and environmental effects in isolation, overlooking the possibility of interactions between genotype and environment [20] . Such interactions might arise if host environment determines whether a microbe colonizes the gut, and genotype determines whether or not that microbe is tolerated or eliminated. The environmental effect would then only be detectable in the subset of hosts whose genotype permits microbe persistence, resulting in a genotype*environment interaction. For example, an important environmental variable, diet, serves as both a source of colonizing bacteria [21] and alters the gut nutritional environment [17] , and so has been shown in many studies to affect the composition of the gut microbiota [13] , [14] , [15] , [16] , [17] . Sex, a genetic trait, also influences the gut microbiota [11] , [21] , [22] , [23] , through poorly understood mechanisms [22] apparently including hormone–microbe interactions [23] , [24] and sex-specific immune responses. If the microbes that respond to sex are also influenced by diet, we might expect to see diet effects that differ between males and females. However, such sex*diet interactions have not been reported so far. Within many natural populations, co-occurring individuals consistently consume different foods [25] . We took advantage of within-population diet variation to test whether diet and sex jointly affect microbiota composition in wild populations of two vertebrates. Such within-population comparisons permit correlative studies of diet-microbiota associations in a natural setting, without the complicating effects of geographic heterogeneity, admixture between disparate populations, potentially misleading effects of artificial laboratory diets and environments, or having to compare different species that differ in many respects. Here we show that natural diet variation is associated with microbial composition within single populations of each of two fish species, the threespine stickleback ( Gasterosteus aculeatus ) and Eurasian perch ( Perca fluviatilis ). These species are intensively studied examples of intraspecific diet variation [26] , [27] , [28] , [29] , [30] , [31] . We supplement these correlative studies with experimental evidence that diet and sex interactively affect microbiota composition in laboratory populations (stickleback and lab mice). Finally, we show that the sex*diet interactions found here also occur in humans. Our results show that across four disparate vertebrate species, diet has a sex-specific effect on host gut microbiota. Consequently, researchers and clinicians need to consider environment by genotype interactions in microbial research and in designing dietary therapies for dysbiosis. We measured the associations between gut microbiota and sex and diet, within two natural fish populations: threespine stickleback from a lake in British Columbia, Canada, and Eurasian perch from a lake in Sweden. Each lake contains a single panmictic population of the respective species. We characterized each individual’s gut microbiota via Illumina sequencing of the V4 region of bacterial 16S rRNA [32] ( Supplementary Data 1 ). We found substantial among-individual variation in microbiota composition within each host population ( Fig. 1 ). For instance, in stickleback the phylum Proteobacteria ranges from <1% of an individual’s microbiome, to over 98% in another individual. Our goal is to evaluate whether individual diet variation and sex contribute to this among-individual microbial heterogeneity. Remarkably, despite this variation among related individuals from the same population, there was substantial conservation in gut microbiota composition between stickleback and perch ( Fig. 2 ), whose lineages diverged ~50 million years ago [33] . 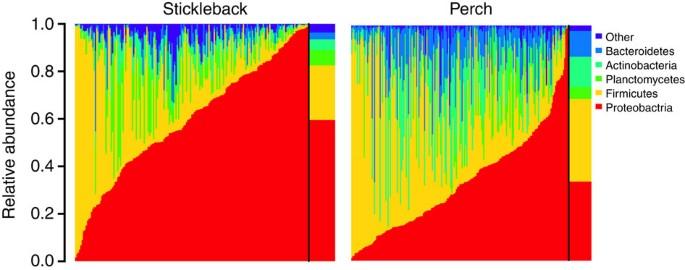Figure 1: There is substantial among-individual heterogeneity in gut microbiota composition within stickleback and perch populations. Columns represent the relative abundance of microbial phyla within individual hosts, and population mean abundance to the right of the black line. In stickleback, Proteobacteria ranged from 1.6 to 98.9% of individuals’ microbiota (mean=57%; 1.1–99.8% in perch). Similar among-individual variation is observed at lower taxonomic ranks (for example, among classes within a phylum). This heterogeneity among individuals is particularly striking, given the strong similarity in mean microbiota composition between stickleback and perch (Fig. 2). Figure 1: There is substantial among-individual heterogeneity in gut microbiota composition within stickleback and perch populations. Columns represent the relative abundance of microbial phyla within individual hosts, and population mean abundance to the right of the black line. In stickleback, Proteobacteria ranged from 1.6 to 98.9% of individuals’ microbiota (mean=57%; 1.1–99.8% in perch). Similar among-individual variation is observed at lower taxonomic ranks (for example, among classes within a phylum). This heterogeneity among individuals is particularly striking, given the strong similarity in mean microbiota composition between stickleback and perch ( Fig. 2 ). 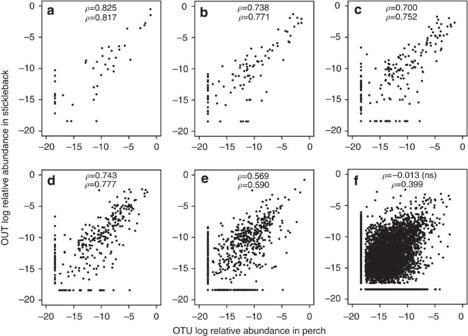Figure 2: Microbial taxon relative abundance is correlated between perch and stickleback. For (a) phyla, (b) classes, (c) orders, (d) families, (e) genera and (f) all OTUs. Spearman rank correlations are provided for each taxonomic level (top value: all taxa, bottom: shared taxa), allP<0.00001 exceptf. To plot taxa absent in one host, a small value was added to all frequencies before log transformation. Complete information on taxonomic composition, relative abundance and prevalence are provided inSupplementary Data 1. Full size image Figure 2: Microbial taxon relative abundance is correlated between perch and stickleback. For ( a ) phyla, ( b ) classes, ( c ) orders, ( d ) families, ( e ) genera and ( f ) all OTUs. Spearman rank correlations are provided for each taxonomic level (top value: all taxa, bottom: shared taxa), all P <0.00001 except f . To plot taxa absent in one host, a small value was added to all frequencies before log transformation. Complete information on taxonomic composition, relative abundance and prevalence are provided in Supplementary Data 1 . Full size image Each population of fish consumes a mixture of substrate-dwelling (littoral) insect larvae and open-water (pelagic) zooplankton. However, within each population individuals differ systematically in their relative use of these resources [28] , [34] , forming a continuum ranging from littoral specialists, through generalists with a mixed diet, to pelagic specialists. Sampling from these ecologically variable populations, we measured carbon and nitrogen stable isotope ratios (δ 13 C and δ 15 N) from each individual, which reflect individuals’ long-term diet. These isotopic measures are widely used to study diet in natural populations [35] . Using isotope ratios of primary littoral and pelagic consumers (mussels and snails) as endpoints, we calculated each individual’s proportional use of littoral carbon ( α ), and trophic position ( tpos ) [36] . Stickleback and perch both exhibited unimodal diet variation: the stickleback population included individuals using as little as 12% to as much as 100% littoral carbon (5–67% in perch), spanning almost a full trophic level ( Supplementary Fig. 1 ). As these host species eat a similar littoral/pelagic continuum of foods and have similar microbiota ( Fig. 2 ), we can test whether diet has similar effects on microbiota in both host species. We took two complementary approaches to assaying diet–microbiota associations. First, we use multivariate methods (Principal Coordinate Analysis (PCoA)) to quantify major axes of microbial variation among individuals, and use these PCoA axes to test for whole-microbiota responses to diet and sex. Second, to explain these whole-microbiota responses we assay whether diet and sex jointly alter the relative abundance of individual microbial taxa (‘operational taxonomic units’ or OTUs). Multivariate analyses of sex and diet effects on microbiota We quantified among-individual variation in gut microbial community composition using PCoA of matrices that contain phylogenetically weighted (UNIFrac) distances between all combinations of individuals. We then used a multivariate analysis of covariance to test whether a matrix of major PCoA axes depended on diet, sex or a sex*diet interaction. Stickleback diet (proportion littoral carbon, α ) had a significant effect on the microbiota ( P =0.041), although diet effects differed between males and females (sex* α , P =0.042). There was no main effect of sex ( P =0.1; Supplementary Fig. 2 ), consistent with weak sex effects in other vertebrates [11] , [15] , [37] . Notably, diet effects were not observed in statistical models that ignored sex*diet interactions ( P >0.7). Perch also exhibited sex-dependent diet effects on PCoA axes (sex* α , P =0.031, sex* tpos P =0.018), whereas diet effects were undetectable when the interaction with sex was omitted. As sex is genetically determined in both stickleback [38] and perch [39] , these sex*diet interactions represent an instance of a genotype-by-environment interaction affecting microbiota composition. Our multivariate analysis of covariance results were further supported by a complementary approach: canonical correlation analysis (CCA) identifies linear combinations of multiple predictor variables that exhibit a multivariate correlation with a linear combination of dependent variables. CCA confirmed that a combination of host traits ( α , tpos and trophic morphology) is correlated with microbiota composition (a combination of PCoA axes). For this analysis, we also include morphological traits associated with feeding (gill raker length and number, body size and gape width [29] ) in the CCA, to test whether diet–microbe associations arise merely from joint correlation with morphology. We find significant canonical correlations between host traits and microbiota in the stickleback population as a whole, and within each sex separately ( P <0.008 within each sex; Supplementary Fig. 3 and Supplementary Data 2 ). Crucially, the major axes of traits and microbes underlying this correlation in males are unrelated to the trait–microbe combinations in females ( Supplementary Fig. 4 ). The canonical correlation axes that best predict microbiota composition rely mostly on isotopic metrics of diet ( Supplementary Fig. 4A ) rather than morphology. Consequently, CCA with only isotopic data yields qualitatively equivalent results. Diet affects relative abundance of microbe OTUs in the wild To identify microbe–diet combinations underlying the multivariate associations described above, we used quasibinomial general linear models (GLMs; see Supplementary Methods for details) to test for diet and sex effects on the abundance of each abundant microbial species (OTUs). Binomial GLMs test whether binomially distributed dependent variables (for example, number of a given OTU sequences out of the total number of reads per host) depend on predictor variables, using a logit transformation to adjust for the heteroscedasticity inherent in binomial data. GLMs allow one to model the relative abundance of a microbe OTU while accounting explicitly for variation in sequence depth across hosts. However, microbe relative abundances are typically overdispersed (more variance than expected with a binomial random variable); hence, we use a more flexible but less powerful quasibinomial model that is less sensitive to outliers and overdispersion. The GLMs address three questions: (i) does OTU abundance depend on diet within each species (and within each sex within each species)? If so, is the size and direction of diet effects conserved (ii) across host species, and (iii) between sexes within species? We focus on abundant microbes (OTUs with at least 0.01% relative abundance, N =516). A small but non-negligible number of microbial OTUs covaried significantly with host diet. Examples of these diet effects are shown in Fig. 3 , chosen to illustrate various patterns of diet, sex and species effects. For instance, intake of littoral carbon ( α ) was significantly associated with altered abundance of 9% of abundant OTUs in stickleback and 14.3% of OTUs in perch ( Fig. 4 ). These percentages of significant α effects are significantly greater than the 5% expected due to false positives alone ( P <0.001), and more than half remain significant after false discovery rate (FDR) corrections ( q <0.05). Likewise, trophic position affects the abundance of 11.1% and 16.6% of OTUs in stickleback and perch, respectively. Analyses of morphology (size, gape width, gill raker length and number, which are all correlated with diet in the two populations) yield similarly widespread significant effects on OTU relative abundances (details not shown). 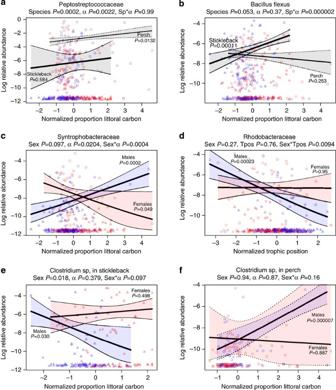Figure 3: Selected examples of microbial OTU responses to diet. Triangles and open circles represent stickleback and perch, respectively. Red/blue indicates females and males. Lines represent quasibinomial GLM estimates with confidence intervals (coloured by sex, grey if combining sexes). GLM estimates ofP-values for model terms are included next to trend lines or in panel headings. Headings indicate the lowest known taxonomic identity of the OTU. OTUs presented here were chosen to illustrate several distinct patterns: (a) overall effect ofαin both host species for an OTU in the Peptostreptococcaceae. There is also a host species effect (P=0.0002), but no interaction effects as diet has parallel (albeit not equally significant) effects in each host. Overall, 11.3 % of abundant OTUs exhibited a main effect ofαacross both hosts (11.5% fortpos). This represents a unique demonstration that environmental effects on the microbiota can be (weakly) extrapolated from one host species to another. (b) A species-specific effect of carbon source onBacillus flexusabundance in stickleback but not perch, underlying a significant species*diet interaction (P=0.0001). This OTU also exhibits a sex*species interaction becauseB. flexusis more abundant in stickleback males than in females (P=0.000014), whereas it shows a nonsignificant tendency to be more abundant in female than male perch (P=0.0954). Neither species exhibits a significant sex*αinteraction. (c) A sex-specific carbon effect on a Syntrophobacteraceae OTU, which is more abundant in littoral males (P=0.049) and in pelagic females (P=0.0002) regardless of host species. (d) Sex-specific trophic position (tpos) effect in which a Syntrophobacteraceae OTU is more common in low trophic position males (P=0.00023), regardless of host species, but is insensitive to trophic position in females (P=0.95). (e,f) A sex*carbon*species interaction onClostridium spabundance, which exhibits opposite diet effects in male stickleback versus male perch (more common in pelagic male sticklebackP=0.03, and in littoral male perchP=0.000007), but is independent of female diet in both hosts. Figure 3: Selected examples of microbial OTU responses to diet. Triangles and open circles represent stickleback and perch, respectively. Red/blue indicates females and males. Lines represent quasibinomial GLM estimates with confidence intervals (coloured by sex, grey if combining sexes). GLM estimates of P -values for model terms are included next to trend lines or in panel headings. Headings indicate the lowest known taxonomic identity of the OTU. OTUs presented here were chosen to illustrate several distinct patterns: ( a ) overall effect of α in both host species for an OTU in the Peptostreptococcaceae. There is also a host species effect ( P =0.0002), but no interaction effects as diet has parallel (albeit not equally significant) effects in each host. Overall, 11.3 % of abundant OTUs exhibited a main effect of α across both hosts (11.5% for tpos ). This represents a unique demonstration that environmental effects on the microbiota can be (weakly) extrapolated from one host species to another. ( b ) A species-specific effect of carbon source on Bacillus flexus abundance in stickleback but not perch, underlying a significant species*diet interaction ( P =0.0001). This OTU also exhibits a sex*species interaction because B. flexus is more abundant in stickleback males than in females ( P =0.000014), whereas it shows a nonsignificant tendency to be more abundant in female than male perch ( P =0.0954). Neither species exhibits a significant sex* α interaction. ( c ) A sex-specific carbon effect on a Syntrophobacteraceae OTU, which is more abundant in littoral males ( P =0.049) and in pelagic females ( P =0.0002) regardless of host species. ( d ) Sex-specific trophic position (tpos) effect in which a Syntrophobacteraceae OTU is more common in low trophic position males ( P =0.00023), regardless of host species, but is insensitive to trophic position in females ( P =0.95). ( e , f ) A sex*carbon*species interaction on Clostridium sp abundance, which exhibits opposite diet effects in male stickleback versus male perch (more common in pelagic male stickleback P =0.03, and in littoral male perch P =0.000007), but is independent of female diet in both hosts. 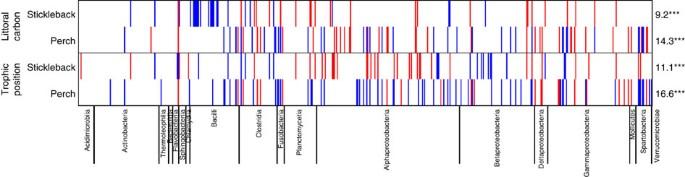Figure 4: Widespread effects of diet on relative abundances of microbe OTUs in perch and stickleback. Rows represent different diet effects (proportion littoral carbon or trophic position) in each of the two host species. Each column in the heatmap represents one of the 566 abundant OTUs (averaging >0.01% relative abundance), arranged by taxonomic group (names of Classes are provided along the bottom of the figure). Thin vertical red bars indicate OTUs whose relative abundance decreases significantly (P<0.05) with the diet metric in a quasibinomial GLM for the focal host species. Blue bars indicate OTUs whose relative abundance increases with the diet metric. On the right side of the figure, we indicate the percentage of the abundant OTUs that exhibit significant main effects of diet within each host species. Asterisks indicate whether this percentage significantly exceeds the 5% expected from false positives (***P<0.001). Full size image Figure 4: Widespread effects of diet on relative abundances of microbe OTUs in perch and stickleback. Rows represent different diet effects (proportion littoral carbon or trophic position) in each of the two host species. Each column in the heatmap represents one of the 566 abundant OTUs (averaging >0.01% relative abundance), arranged by taxonomic group (names of Classes are provided along the bottom of the figure). Thin vertical red bars indicate OTUs whose relative abundance decreases significantly ( P <0.05) with the diet metric in a quasibinomial GLM for the focal host species. Blue bars indicate OTUs whose relative abundance increases with the diet metric. On the right side of the figure, we indicate the percentage of the abundant OTUs that exhibit significant main effects of diet within each host species. Asterisks indicate whether this percentage significantly exceeds the 5% expected from false positives (*** P <0.001). Full size image These diet effects were disproportionately concentrated in certain microbial clades ( Fig. 4 ). For example, in stickleback α effects were found in 36% of Bacilli OTUs, 25% of Sphingobacteriia and 21% of Clostridia (χ 2 =56.37, P <0.001). In perch, α was associated with changed abundance of 66% of Fusobacteria, 54% of Spartobacteria, 40% of Deltaproteobacteria, 21% of Clostridia and 18% of Alphaproteobacteria ( χ 2 =60.83, P <0.001). Significant effects of tpos were more evenly spread among stickleback microbial clades ( χ 2 =27.64, P =0.230), but in perch tpos effects were concentrated in Fusobacteria (66% of OTUs), Spartobacteria (46%), Deltaproteobacteria (40%), Alphaproteobacteria (20%), and Clostridia and Betaproteobacteria (both 18%; χ 2 =54.97, P <0.001). To evaluate the functional significance of varying OTU relative abundance, we used 16S sequences to indirectly infer microbiome gene composition using PICRUSt [40] . Despite inherent limitations in predicting genic composition of poorly known microbes from wild fish, we found that the abundance of inferred gene ontology (GO) categories varied with stickleback diet ( Supplementary Fig. 5 ). For instance, the strongest effects include a trend towards fewer vitamin and energy metabolism genes in stickleback with higher trophic positions, consistent with different nutritional intakes. Unfortunately, little is known about the biochemical composition of the natural prey, preventing mechanistic interpretation of the diet–GO associations. Future progress will require manipulation of specific dietary nutrients and finer-resolution GO definitions. Different host species exhibit similar diet effects We next tested whether stickleback and perch exhibit similar diet effects on OTU relative abundance. Each abundant OTU was tested for dependence on diet ( α and tpos ), sex, host species and interactions between these variables, using quasibinomial GLMs, including all wild-caught fish specimens together in one analysis per OTU. When we find a main effect of diet and no significant species*diet interaction, we may infer that the OTU responds to a littoral or pelagic diet in a similar manner in stickleback and in perch (for example, Fig. 3a ). Across both host species, 11.3% of shared OTUs exhibit significant main effects of littoral carbon, and 11.5% of OTUs show main effects of trophic position. Roughly half of these remain significant after FDR correction (5.6% and 6.7% for α and tpos , respectively). In contrast, fewer shared OTUs exhibit species* α or species* tpos interactions (6.9% and 5.1%, not significantly >5% FDRs), although 4% of OTUs do exhibit species*diet interactions after FDR correction indicative of species-specific responses to diet. We infer that effects of littoral carbon intake and trophic position are similar in these two geographically and evolutionarily very divergent host species. This conclusion is confirmed by a significant positive correlation between diet effects on OTUs in stickleback and diet effects on the same OTUs in perch ( Table 1 ). Table 1 Comparisons of the effect size* of diet on gut microbial OTUs, in different host groups (species, sex, or treatment) † . Full size table Experimental diet manipulation alters gut microbiota Confirming the causal effect of diet on microbiota composition, captive male stickleback experimentally fed littoral or pelagic prey exhibited divergent microbiota (multivariate analysis of variance (MANOVA) of diet effect on weighted or unweighted PCoA axes, P <0.0001; Fig. 5 ). In this experiment, we focus exclusively on males to establish the causal effect of diet on microbiota without confounding effects of sex, or reproductive state: all males were nesting at the time of sampling, whereas it is harder to ensure all females are simultaneously in the same reproductive state (for example, all equally gravid). The microbial discriminant axis that best distinguishes chironomid- from Daphnia -fed stickleback is associated with changes in both the presence/absence and relative abundance of various microbial taxa (examples in Supplementary Fig. 6 ). These changes in microbial composition coincided with changes in relative abundance of GO functions, inferred indirectly from 16S sequences using PICRUSt [40] . Daphnia -fed fish carried fewer genes involved in energy metabolism ( P <0.0001), cofactor/vitamin metabolism ( P <0.0001), translation ( P =0.0007), replication and repair ( P =0.0013), cell communication ( P =0.0051), nucleotide metabolism ( P =0.0148), excretory system ( P =0.0209) and more genes involved in signal transduction ( P <0.0001), digestive system (0.0040), infectious disease ( P =0.0101), carbohydrate metabolism ( P =0.0176) and transcription ( P =0.0434). Of these, a few GO categories were found to respond to diet in the wild stickleback as well (cofactor/vitamin metabolism, signal transduction and energy metabolism; Supplementary Fig. 5c ). From the little that is known about Daphnia and chironomid nutritional value, chironomids contain more protein and less carbohydrate per unit dry mass and there are only modest quantitative differences in amino acid and lipid composition between the prey [41] , [42] . These quantitative, rather than qualitative, differences make it difficult to interpret the functional value of the divergence in microbial GO composition. However, from the available (albeit indirect) data it does appear that dietary changes in microbiota probably alter metagenomic function. Further studies will be required to identify the functional relationship between these GO changes and prey nutrient content. 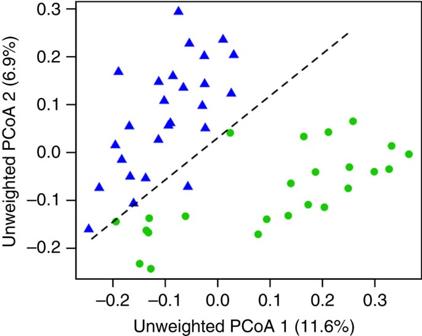Figure 5: Experimentally manipulated diet alters gut microbiota composition in captive threespine stickleback. Differences in microbiota composition (unweighted PCoA axes 1+2) between male stickleback fed littoral versus pelagic prey. Daphnia-fed fish are indicated by blue triangles, chironomid-fed fish are green circles. The percentages in the axis labels indicate the percentage of total variation in microbial community structure that is associated with each PCoA axis. A dashed line separates the two treatments to emphasize the nearly non-overlapping differences between diet treatments. A MANOVA confirmed that unweighted PCoA axes 1–12 (top 50% of variation) exhibit a significant association with diet (P=0.00004), but not tank (P=0.283). Similar effects were observed for weighted PCoAs (dietP=0.000002; tankP=0.889). Figure 5: Experimentally manipulated diet alters gut microbiota composition in captive threespine stickleback. Differences in microbiota composition (unweighted PCoA axes 1+2) between male stickleback fed littoral versus pelagic prey. Daphnia-fed fish are indicated by blue triangles, chironomid-fed fish are green circles. The percentages in the axis labels indicate the percentage of total variation in microbial community structure that is associated with each PCoA axis. A dashed line separates the two treatments to emphasize the nearly non-overlapping differences between diet treatments. A MANOVA confirmed that unweighted PCoA axes 1–12 (top 50% of variation) exhibit a significant association with diet ( P =0.00004), but not tank ( P =0.283). Similar effects were observed for weighted PCoAs (diet P =0.000002; tank P =0.889). Full size image Lab-reared fish carried few naturally occurring OTUs ( Supplementary Fig. 7a ). Focusing on the subset of OTUs that were present in both wild and captive stickleback, the OTUs that were more abundant in littoral wild fish were not generally the same as OTUs enriched in lab fish fed littoral prey (chironomids). As a result, there was no correlation between littoral/pelagic diet effects on OTUs in the lab versus wild ( Supplementary Fig. 7b ). The difference between lab-reared and wild fish presumably reflects some unknown feature of their respective environments (water microbiota, water chemistry, different prey nutrients or microbiota) or different host genotypes. Whatever the mechanism underlying this difference, our finding illustrates a broader point that laboratory studies, which are clearly necessary for fully controlled manipulative experiments, generally do not recreate natural environments and microbiota. Consequently, laboratory studies of host–microbiota associations should carefully consider what aspects of their results can be generalized to natural populations. Sexes do not exhibit similar diet effects in the wild Although the distantly related host species exhibited similar (positively correlated) diet effects on OTUs, the same was not true for sexes within each host species. There is some dietary divergence between sexes within each host species. However, the range of male and female stickleback α -values overlaps by 66% and overlap for tpos is even higher (86%). Consequently, using just α (or tpos ), one would misclassify 25% (33%) of individuals to the wrong sex. Diet overlap between the sexes is higher in perch (90.4% and 91.7%). Because of this dietary overlap between the sexes, we can use GLMs to statistically partition sex versus diet effects on each OTU’s abundance, and to test for a sex*diet interaction. An interaction would imply that diet has different effects (slopes) in males and females. In the quasibinomial GLMs with diet, sex, species and all interaction effects, diet effects were often sex specific ( Fig. 3c–f ). Almost as many OTUs exhibited sex-specific diet effects (indicated by sex*diet interactions), as the number of OTUs that exhibited main effects of diet. Sex* α interactions were significant in 8.1% of abundant stickleback OTUs ( Fig. 6 ) and sex* tpos in 7.2% of perch OTUs. Both percentages significantly exceed false positive expectations and include FDR-robust results ( q <0.05 for >4% of OTUs per comparison). In contrast, sex* α interactions in perch and sex* tpos interactions in stickleback were slightly less common (6.1% and 5.7%, respectively). Although these were only slightly (and not significantly) above the 5% null expectation, these counts do include OTUs whose diet effects remained significant after FDR correction ( q <0.05, 2.6% and 2.8% of OTUs, respectively). 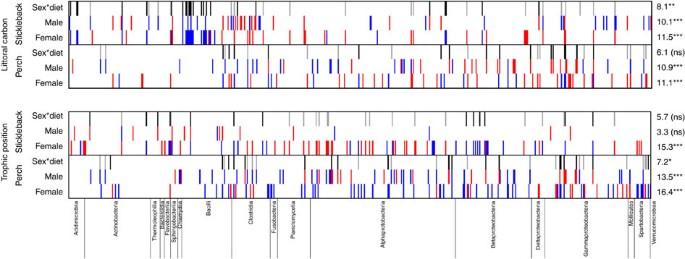Figure 6: The relative abundances of some microbial OTUs depend on an interaction between sex and diet, in both perch and stickleback. The top heatmaps represent how OTUs covary with host individuals’ proportional reliance on littoral carbon (α). The bottom heatmaps represent the effects of host trophic position on OTU abundance. Each column represents one of the 566 abundant OTUs (averaging >0.01% relative abundance), arranged by taxonomic group (names of classes are provided along the bottom of the figure). Within each heatmap, rows with red/blue bars indicate the effect of a given diet measure on individual OTUs for (from top to bottom) male stickleback, female stickleback, male perch and female perch. Thin vertical red bars indicate OTUs whose relative abundance decreases significantly (P<0.05) with the diet metric in a quasibinomial GLM for the focal host species and sex. Blue bars indicate OTUs whose relative abundance increases with the diet metric (a ‘positive’ effect). For each diet measure and species, we also include a row indicating OTUs with significant sex*diet interaction effects in the GLM. Black bars represent OTUs with more positive diet effects in females than males. This can arise, for example, when (i) an OTU is more abundant in hightposfemales (positive effect) and unresponsive totposin males (no effect), (ii) when an OTU is unresponsive totposin females (no effect) but decreases withtposin males (negative effect), or (iii) when an OTU changes withtposin both sexes but exhibits a more positive slope in females. Grey bars represent OTUs with more positive diet effects in males than females. On the right side of the figure, we indicate the percentage of the abundant OTUs that exhibit significant main effects of diet within each host sex/species combination, or that exhibit sex*diet interactions. Asterisks indicate whether this percentage significantly exceeds the 5% expected from false positives (*P<0.05; **P<0.01; ***P<0.001). Figure 6: The relative abundances of some microbial OTUs depend on an interaction between sex and diet, in both perch and stickleback. The top heatmaps represent how OTUs covary with host individuals’ proportional reliance on littoral carbon (α). The bottom heatmaps represent the effects of host trophic position on OTU abundance. Each column represents one of the 566 abundant OTUs (averaging >0.01% relative abundance), arranged by taxonomic group (names of classes are provided along the bottom of the figure). Within each heatmap, rows with red/blue bars indicate the effect of a given diet measure on individual OTUs for (from top to bottom) male stickleback, female stickleback, male perch and female perch. Thin vertical red bars indicate OTUs whose relative abundance decreases significantly ( P <0.05) with the diet metric in a quasibinomial GLM for the focal host species and sex. Blue bars indicate OTUs whose relative abundance increases with the diet metric (a ‘positive’ effect). For each diet measure and species, we also include a row indicating OTUs with significant sex*diet interaction effects in the GLM. Black bars represent OTUs with more positive diet effects in females than males. This can arise, for example, when (i) an OTU is more abundant in high tpos females (positive effect) and unresponsive to tpos in males (no effect), (ii) when an OTU is unresponsive to tpos in females (no effect) but decreases with tpos in males (negative effect), or (iii) when an OTU changes with tpos in both sexes but exhibits a more positive slope in females. Grey bars represent OTUs with more positive diet effects in males than females. On the right side of the figure, we indicate the percentage of the abundant OTUs that exhibit significant main effects of diet within each host sex/species combination, or that exhibit sex*diet interactions. Asterisks indicate whether this percentage significantly exceeds the 5% expected from false positives (* P <0.05; ** P <0.01; *** P <0.001). Full size image We next calculated the magnitude of diet effects on each abundant OTU’s relative abundance, within each sex and species. If OTUs tend to respond similarly to diet in males versus females, these effect sizes should be positively correlated. On the contrary, diet effects on OTU abundance in males were uncorrelated with effects in females ( Table 1 ). Sexes also differed in the overall magnitude of diet effects on OTUs, which were significantly stronger in female than male stickleback, and stronger in male than female perch ( Table 1 ). PICRUSt-inferred GO counts also revealed many sex*diet interactions ( Supplementary Fig. 5c ), no significant correlation in diet effects between sexes within each species (all P >0.1) and stronger overall diet effect sizes in female than male stickleback ( t =−6.53, df=37, P <0.0001). Thus, diet effects on gut microbiota cannot be extrapolated from one sex to the other, either in terms of taxonomic composition or inferred gene functions. Sex-specific diet effects in lab-reared stickleback We carried out a second diet manipulation experiment with laboratory stickleback, this time feeding chironomids or Daphnia to both captive male and female stickleback. A MANOVA confirmed that the 21 leading unweighted microbial PCoA axes (accounting for 50% of cumulative among-individual variation) exhibit significant effects of diet ( P =0.001) and a sex*diet interaction ( P =0.042), but not sex ( P =0.473). The sex*diet interaction confirms our findings from wild-caught stickleback (E.D. Fig. 7 ). Using a discriminant function analysis (DFA) to summarize differences between sexes and diets (four groups total; Fig. 7 ), the first discriminant axis is most strongly associated with diet (analysis of variance, diet P <0.0001, sex P =0.0006 and sex*diet P =0.0319). The second axis predominantly reflects the sex-specific nature of diet effects (diet P =0.0125, sex P =0.0029 and sex*diet P <0.0001). 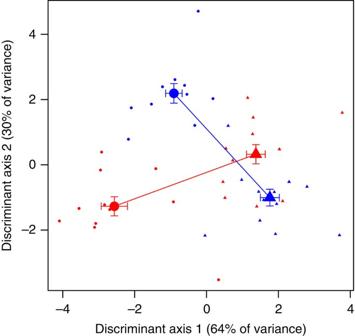Figure 7: Microbiota exhibit different responses to diet in captive male and female stickleback. We obtained gut microbial DNA from lab-reared stickleback fed chironomids (15 females, 13 males) andDaphnia(14 females, 13 males). We obtained a total of 5,226,827 sequence reads from 15 females (red points) and 13 males (blue points) experimentally fed chironomids (circles), and 14 females and 13 males fedDaphnia(triangles). We averaged 54,446 sequence reads per sample (range: 406–299,947; mean of 31,409), identified as 1,460 microbial OTUs. Here we plot individuals’ scores along the first two linear DFA of microbiota composition (unweighted PCoA axes 1–21) that separate groups (combinations of sex and diet). Larger points with s.e. bars indicate group means. Within each sex, lines represent the diet effect (connecting means forDaphnia- to chironomid-fed fish); the angle between these lines emphasizes the sex-dependent diet effects. In particular, the following taxa are more common inDaphnia-fed males and chironomid-fed females: OTUs in the families Hyphomonadaceae (P=0.0000014), Isosphaeraceae (P=0.00006), Haliangiaceae (P=0.00016), Staphylococcaceae (P=0.0015), Pirellulaceae (P=0.0018), Aeromonadaceae (P=0.0035) and Saprospiraceae (P=0.0036), and in the generaBurkholderia(P=0.000010),Veillonella(P=0.0000012),Staphylococcus(P=0.000018),Stenotrophomonas(P=0.00135) andParacoccus(P=0.0018). Figure 7: Microbiota exhibit different responses to diet in captive male and female stickleback. We obtained gut microbial DNA from lab-reared stickleback fed chironomids (15 females, 13 males) and Daphnia (14 females, 13 males). We obtained a total of 5,226,827 sequence reads from 15 females (red points) and 13 males (blue points) experimentally fed chironomids (circles), and 14 females and 13 males fed Daphnia (triangles). We averaged 54,446 sequence reads per sample (range: 406–299,947; mean of 31,409), identified as 1,460 microbial OTUs. Here we plot individuals’ scores along the first two linear DFA of microbiota composition (unweighted PCoA axes 1–21) that separate groups (combinations of sex and diet). Larger points with s.e. bars indicate group means. Within each sex, lines represent the diet effect (connecting means for Daphnia - to chironomid-fed fish); the angle between these lines emphasizes the sex-dependent diet effects. In particular, the following taxa are more common in Daphnia -fed males and chironomid-fed females: OTUs in the families Hyphomonadaceae ( P =0.0000014), Isosphaeraceae ( P =0.00006), Haliangiaceae ( P =0.00016), Staphylococcaceae ( P =0.0015), Pirellulaceae ( P =0.0018), Aeromonadaceae ( P =0.0035) and Saprospiraceae ( P =0.0036), and in the genera Burkholderia ( P =0.000010), Veillonella ( P =0.0000012), Staphylococcus ( P =0.000018), Stenotrophomonas ( P =0.00135) and Paracoccus ( P =0.0018). Full size image Of the 241 abundant OTUs found in this experiment, 42 (17.4%) exhibited significant sex*diet interactions in quasibinomial GLMs and 14 remained significant following FDR correction ( q <0.05). In all instances of significant sex*diet interactions, the interaction reflects a significant diet effect in one sex and a nonsignificant diet effect in the other sex (for example, Supplementary Fig. 8 ), rather than significant opposing effects. However, in contrast to the wild-caught fish we did find a significant positive correlation between how diet affected OTU abundance in males, versus how the same diet affected OTU abundance in females. This shows that diet effects can be extrapolated between sexes in an artificial laboratory setting, but even there the correlation is weak ( r =0.17, P =0.008; Supplementary Fig. 9 ). Only three of 241 abundant OTUs exhibit significant diet-induced shifts in abundance in the same direction in both males and females. Despite this positive correlation, the significant sex*diet interactions (for PCoAs and for individual OTUs) confirms our finding from wild-caught fish that diet alters the gut microbiota in a sex-dependent manner. Interestingly, the effect of diet on gut microbiota in this experiment is not driven by differential ingestion of food-associated microbes: in a separate study [43] , we compared the microbiota of Daphnia , chironomids and fish fed Daphnia or chironomids, showing that fish gut microbiota do not disproportionately resemble the microbiota of their food. Thus, diet effects reflect differences in gut nutritional environment rather than colonization. Sex*diet interactions also affect mammalian gut microbiota Based on the sex*diet interactions we found in fish, we then tested for sex-specific diet effects on microbiota of two mammals. In both humans and mice, diet has previously been shown to modify the gut microbiota [7] , [13] , [14] , [15] , but the possibility of sex*diet interactions has been overlooked. Re-analysis of published human data [15] showed sex*diet interactions affecting the abundance of a significant fraction of the 125 most abundant OTUs (for example, Supplementary Fig. 10 ). We used principal component analysis to quantify major dimensions of diet variation in humans (see Supplementary Data 3 for loadings of diet variables), retaining the top nine diet principal component (PC) axes whose eigenvalues exceeded broken-stick model expectations. Six of the top nine dietary PC axes exhibited a significant excess of significant sex*diet interactions ( Supplementary Data 3 ). Sex*diet interactions are particularly common among OTUs in the Fusobacteriaceae (60% of which show significant interaction effects), significantly more often than seen in other families. Diet effects on OTUs in males were uncorrelated with diet effects in females for seven out of these nine major diet axes ( Table 1 and Fig. 8a ), although for diet PC axes 2 and 3 (12.6% and 6% of diet variance, respectively) male and female microbiota exhibited weakly correlated diet effects ( Fig. 8b ). Despite the correlated response to diet PC2 in males and females, only two OTUs responded significantly and in the same direction to male and female PC2 score: a Lachnospiraceae sp and a Bacteroides sp. were consistently more common in diets with low saturated fats and high fibre. Unlike stickleback and perch, we found no significant tendency for diet effects in humans to be stronger in one sex than the other, although the trend is consistent (males having larger diet effects) for all ten PC axes. In conclusion, whereas the typical approach to studying diet effects on the microbiota has been to assume such effects hold in both sexes (assuming a correlation ρ ≈1), we find such correlations are weak at best. 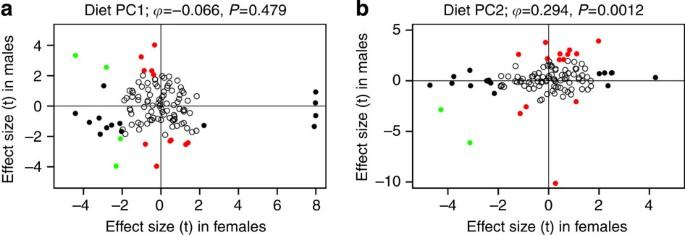Figure 8: Comparison between male and female diet effects on the human gut microbiota. Diet is measured here by the top two principal component axes of detailed nutritional data from Wuet al.15, seeSupplementary Data 3for PC loadings to interpret these axes. Diet effects are uncorrelated (A: diet PC1) or weakly positively correlated (B: diet PC2) between males and females. Each point represents the female and male diet effect on one of the 125 most abundant OTUs (>0.1% mean relative abundance). Diet effect is measured as at-statistic, scaling the slope of OTU relative abundance versus diet PC score (calculated in a sex-specific quasibinomial GLM), by the s.e. of that slope. Open points are not statistically significant (P>0.05). Black points are significant in females, red significant in males and green points are significant in both. Horizontal and vertical lines visually distinguish OTUs with positive effect estimates in both sexes (top right quadrant), or negative effects in both sexes (bottom left), or opposite effects in males versus females (top left or bottom right). Spearman rank correlation tests are provided above each panel. Figure 8: Comparison between male and female diet effects on the human gut microbiota. Diet is measured here by the top two principal component axes of detailed nutritional data from Wu et al . [15] , see Supplementary Data 3 for PC loadings to interpret these axes. Diet effects are uncorrelated (A: diet PC1) or weakly positively correlated (B: diet PC2) between males and females. Each point represents the female and male diet effect on one of the 125 most abundant OTUs (>0.1% mean relative abundance). Diet effect is measured as a t -statistic, scaling the slope of OTU relative abundance versus diet PC score (calculated in a sex-specific quasibinomial GLM), by the s.e. of that slope. Open points are not statistically significant ( P >0.05). Black points are significant in females, red significant in males and green points are significant in both. Horizontal and vertical lines visually distinguish OTUs with positive effect estimates in both sexes (top right quadrant), or negative effects in both sexes (bottom left), or opposite effects in males versus females (top left or bottom right). Spearman rank correlation tests are provided above each panel. Full size image Diet manipulation in male and female lab mice (fed high fat versus chow diets) also revealed significant sex*diet interactions after FDR corrections ( Supplementary Fig. 11a and Supplementary Data 4 ). For example, Lactobacillus , Alistipes , Lachnospiraceae and Clostridium were more abundant in males fed a high-fat rather than chow diet, whereas in females these genera were less abundant in high-fat diets. Despite a handful of such sex*diet interactions, in general microbes exhibited similar responses to male versus female diets, as illustrated by a positive correlation between male and female diet effect sizes ( r =0.746, P <0.001, Supplementary Fig. 11b ). Thus, lab mice are an exception to the sex-specific diet effects that we found in stickleback, perch and humans. The fact that we do find significant between-sex correlations for lab mice (and to a lesser extent in lab stickleback and some human diet axes) confirms the utility of this analytical approach, and makes the lack of such correlations in wild fish and in humans (for most diet axes) all the more striking. It is widely accepted now that vertebrates’ diet modulates the species composition of their symbiotic gut microbiota [15] , [17] . However, most studies of dietary control of microbiota have either been conducted on populations fed non-natural diets (for example, laboratory mice, zebrafish and arguably humans) [44] , or comparing disparate species [13] . We took advantage of naturally occurring within-population diet variation in two species of fish to test for diet–microbiota correlations. This represents one of only a very few studies, to date, of gut microbial variation within wild vertebrate populations. Our study showed, first, that there is substantial among-individual variation in gut microbial composition in natural populations. Second, we found that individual diet explained some of this microbial variation among individuals. Third, and more profoundly, we found that diet effects are largely sex specific. Whether we examine microbial PCoA axes, or individual OTUs, there is a widespread tendency for diet effects on microbiota, when they exist, to be different in males versus females. This entails both differences in effect direction and magnitude. For instance, knowing whether a microbe increased/decreased with a more littoral diet in female stickleback conferred no information about how that microbe responded to littoral diet in male stickleback (effects were uncorrelated). Moreover, microbes systematically responded more strongly to the diet of stickleback females than the diet of males. As sex is genetically determined in both fish species studied here, this represents a rare instance of a genotype-by-environment interaction regulating the gut microbiota. Due to this interaction, we cannot reliably generalize diet effects observed in one sex to the other sex of the same species. Laboratory diet manipulations in stickleback also revealed sex-specific diet effects, although there was some weak correlation between male and female diet effects in this more controlled setting. The sex-specific effects are particularly surprising given that very distantly related host species (stickleback and perch) exhibited correlated diet effects on microbial OTUs, whereas sexes within the same species exhibited uncorrelated diet effects. The generally sex-specific diet effects on the human microbiome further supports our results from wild and lab fish. The one strong counter-example to these sex-specific effects comes from laboratory populations of mice fed highly simplified diets, where males and females exhibited generally similar diet effects. We are cautious about comparing this positive correlation with the results from wild stickleback, perch and humans, because lab mice have been maintained in highly artificial environments for many generations and so may be unrepresentative of natural populations. Indeed, comparing wild versus laboratory stickleback, we found that microbial taxa showing diet (or sex*diet) effects in the lab were not the same as the taxa showing diet (or sex*diet) effects in the wild [43] . The mechanistic basis of these diet effects remains unclear. In both lab and wild stickleback, diet was associated with changes in the relative abundance of OTUs and inferred GO categories. An important caveat is that these counts of GO categories are indirect, inferred from 16S sequences and the GO gene composition of known microbe genomes. The microbiota of wild fish may be sufficiently different from these known genomes to cause inaccurate estimates of GO composition. However, at present this represents our best available evidence that diet effects on the microbiome may have consequences for host metabolism and digestion. Unfortunately, too little is known about prey nutritional composition and stickleback nutritional needs to clearly link changes in GO composition to changes in nutritional inputs or host requirements. The mechanisms underlying sex modulation of diet effects are similarly uncertain. Studies in mammals have shown that sex hormones can modulate microbiota composition [23] , [24] . In addition, mucosal immune function and susceptibility to inflammatory bowel diseases differs between sexes [24] , [45] , [46] , [47] . At first glance, it would seem that such sex effects should generate systematic microbial differences between males and females (main effects of sex in our statistical models), which are relatively rare in our data sets. However, if sex hormone-dependent microbes are also affected by host diet, then interactions are possible. As a hypothetical example, consider a microbe taxon that is more strongly suppressed by the male mucosal immune system, and requires a particular nutrient to proliferate. Within males, the microbe would be rare or absent regardless of diet, but diet effects would be observed in immunologically more tolerant females, resulting in a sex*diet interaction. Our findings do not at present identify the mechanisms driving either sex or diet effects. Instead, we show for the first time that sex and diet do interactively control microbiota composition, highlighting an urgent need to identify and explain both types of mechanisms and how they interact. Host sex hormones and sex differences in immune function seem probable places to begin such investigations [23] , [24] . More generally, our results represent an example of microbiota depending on an interaction between environment and genotype, sex being just one of many possible genetic polymorphisms that could modulate environmental effects. This represents one of the first studies we are aware of to demonstrate such an interaction. This finding is likely to have practical consequences. First, studies of gut microbiota should habitually account for sex (and its interactions with other factors) even when there is no main effect of sex. Studies that fail to account for sex [11] , [48] , [49] will overlook these interactions and may consequently fail to detect major environmental influences on the gut microbiota, such as diet or drug effects. Second, we propose that sex-specific environmental effects might contribute to the sex-biased rate of some diseases associated with dysbiosis, such as inflammatory bowel diseases [24] . Finally, there is fast-growing interest in changing host environment (diet, stress, drugs) to achieve therapeutic changes in microbiome composition that might prevent or alleviate diseases arising from dysbiosis [19] , [50] . If genotype-by-environment interactions prove to be common in diverse host species, as our results suggest, then therapeutic changes to the environment will not work equally well for all host genotypes, or in both sexes. Consequently, treatment of microbially associated diseases might need to account for these interactions, potentially requiring therapies tailored to host sex and possibly other aspects of host genotype. Sampling from natural populations In June 2008, we set unbaited minnow traps in Cedar Lake on Vancouver Island, British Columbia (50°12′09″ N, 125°33′58″ W), capturing 398 stickleback ( Gasterosteus aculeatus ). This lake contains a single phenotypically unimodal and genetically panmictic population. To capture perch ( Perca fluviatilis , N =255), we trapped overnight in Lake Erken, Sweden (59°51′26″N, 18°35′52″E; July 2009) using four survey-link gill nets targeting a full size range. Specimens were immediately frozen at −20 °C and stored at −80 °C in the lab. For each species, fish were captured along a short stretch of (~200 m) lake shore, on a single day, to minimize temporal and spatial heterogeneity in diet and microbiota. Both species were collected in compliance with ethical regulations for use of research animals, with approval by University of Texas Institutional Animal Care and Use Committee (protocol 07100201) and University of Uppsala Animal Testing Ethics Board protocol C80/13. Previous research indicated that within both lakes individuals vary along a continuum from littoral specialists, to dietary generalists, to pelagic specialists [27] , [51] . Note that ‘benthic’ and ‘limnetic’ are sometimes used in place of littoral or pelagic when describing fish ecotypes or feeding strategies. To avoid confusion with genetically divergent pairs of benthic and limnetic fish species found in some lakes, we use littoral/pelagic to describe feeding variation within single populations. Experimental diet manipulations We conducted two stickleback diet manipulation experiments. First, we fed nesting adult males (standardizing reproductive state) either of two foods to confirm that diet alters gut microbiota. After finding sex*diet interactions in the wild, a lab second experiment applied the food treatments to subadult male and female stickleback to test for interactions. Laboratory diet manipulations were covered by the University of Texas Institutional Animal Care and Use Committee protocols 2009-00074 and 2013-000036. We compared the gut microbiota of captive stickleback fed divergent diets. In vitro fertilization yielded 40 families of stickleback derived from wild-caught parents from Roberts Lake, British Columbia (50°12′55″N, 125°32′29″W). Surface-sterilized eggs were transported to the University of Texas, reared separately in 3-l tanks with shared recirculating water on a diet of hatched brine shrimp and trout chow. Eighteen-month-old individuals were mixed to recreate a natural outbred population, then randomized across eight 100-l aquaria. For 2 months, the fish were fed either chironomid larvae (littoral prey) or Daphnia (pelagic prey), four tanks each, with separate non-recirculating water supplies to avoid cross-contamination. To standardize reproductive state, males were isolated in individual tanks and allowed to nest, then held >18 h without food to allow their guts to clear their last meal before euthanasia and microbe sequencing as described below. We next manipulated male and female stickleback diets to test whether diet effects are sex-specific. Using wild-caught stickleback from Gosling Lake (50°03′26″N, 125°30′07″W), we generated fifty full-sib families reared as described above. At age 9 months, we randomly combined fish and split them into Daphnia -fed and chironomid-fed treatments for 4 weeks, then fasted 24 h to clear intestines before sampling gut microbiota. Eighteen HMDP strains of mice [52] , bred at the University of California, Los Angeles, were maintained on a chow diet (Ralston Purina, 18% kcal fat) until age 8 weeks. A subsample of males and females were transitioned to a high-fat, high-sucrose diet HF/HS (Research Diets-D12266B:16.8% kcal protein, 51.4% kcal carbohydrate and 31.8% kcal fat), while male and female control mice were fed chow. We sequenced the microbiota of 56 and 54 male and female HF/HS mice, pooling same-sex, same-diet and same-strain mice before sequencing (average 2 mice/strain, using strains from the Hybrid Mice Diversity Panel, listed in Supplementary Data 5 ). Mice (adults of both sexes) were treated in accordance with ethical regulations, with approval from the Chancellor’s Animal Research Committee for protocol 1992-169-62K. Phenotypic measurements We weighed fish to 0.01 g and used digital calipers to measure morphological traits previously associated with among-individual diet variation in stickleback [29] , [34] , [53] , [54] , [55] : standard length, gape width and gill raker number, and measured the length of the longest gill raker with an ocular micrometer ( Supplementary Data 6 ). Individuals were sexed by inspecting gonads, and the intestine was removed in its entirety and refrozen at −80 °C. A section of caudal penduncle muscle was dried at 55 °C, ground and ≈1 mg was used for carbon and nitrogen stable isotope quantitation at the University of California at Davis Stable Isotope Facility. We also measured isotopes from tissue sampled from mussels (filter-feeding basal pelagic consumers) and snails (epiphytic grazing basal littoral consumer) from each lake. These isotope ratios are widely used to study feeding ecology and nutrient dynamics in wild populations [35] , [36] , [56] , [57] . Carbon isotopes are fixed in different ratios by different primary producers in lakes. As these isotopes are retained in consumers with little fractionation, the isotope ratios measure individuals’ relative reliance on resources that differ in δ 13 C (refs 58 , 59 ). The ratio of 12 C and 13 C is expressed relative to a fixed reference ( Pee Dee Belemnite ): Comparing stickleback δ 13 C with that of mussels and snails, which are primary consumers that represent pelagic and littoral extremes, one can calculate the proportion littoral carbon in an individual fish’s diet [36] : The ratio of 14 N: 15 N is also expressed using delta notation relative to a standard (air). Unlike δ 13 C, δ 15 N increases by ~3.4 δ 15 N per trophic level in fish due to unequal fraction during digestion and assimilation [36] . We can therefore calculate the trophic position of individual fish: where the baseline expectation is: A crucial aspect of stable isotope ecology is that carbon and nitrogen in animals’ tissues turn over slowly. In fish, muscle δ 13 C and δ 15 N have half-lives of several months, averaging over long-term diet, as evidenced by correlations with foraging observations, gut contents and trophic morphology [26] , [29] , [34] , [53] , [54] , [55] , [60] , [61] . Caudal peduncle muscle is readily biopsied with minimal contribution of other tissues. We do not report stomach contents analyses in this study because stickleback and perch prey are sufficiently different such that taxon-based measures of diet and could not be compared across species. Furthermore, we wished to minimize contributions of microbes in recently ingested prey. Current-day stomach contents would be more likely to generate such transient microbial effects, as opposed to isotopic measures of diet that integrate across months of foraging. Amplification and sequencing of bacterial 16S rRNA genes Subsampling from the wild collections, we extracted DNA from intestines (dissected in sterile conditions) from 192 individuals per host species, using the Powersoil DNA Isolation Kit (MO BIO Laboratories, Carlsbad, CA) with the following protocol modifications. After adding Solution C1, the sample was incubated at 65 °C for 10 min followed by only 2 min of vortexing horizontally at maximum speed. The final elution step was performed two times with a volume of 75 μl of Solution C6 each, incubating for 5 min each time before eluting DNA. We obtained DNA from the entire stickleback intestine (~20 mg, much smaller than the 100 mg recommended for the Powersoil Kit), and for perch we used a 100-mg section from the middle of the intestine. We amplified the V4 hypervariable region of the 16S rRNA gene (positions 515 to 806, based on Escherichia coli numbering) using the standard PCR protocol of the Earth Microbiome Project [62] , [63] . The forward PCR oligonucleotide contained the 5′ Illumina sequencing adapter, a 10-nt pad sequence, followed by the 515 16S specific linker-primer sequence (5′-GTGTGCCAGCMGCCGCGGTAA-3′) described in refs 64 , 65 . The reverse primer contained the 3′ reverse complement of the Illumina sequencing adapter, the 12-nt Golay barcode, a 10-nt pad sequence followed by the 16S specific 806R reverse linker-primer (5′-CC GGACTACHVGGGTWTCTAAT-3′). All PCR reactions were performed in triplicate with 1 × ‘5 Prime Hot Master Mix’, 5 pmol forward and reverse primers and 1 μl template DNA per 25 μl reaction. Replicate PCR reactions for each sample were combined and quantified with Picogreen double-stranded DNA reagent to facilitate pooling equimolar amounts of amplicon for sequencing. Negative controls (no sample added) were included in both the DNA extraction and 16S PCR amplification stages to test for contamination; these PCRs yielded negligible DNA concentrations during Picogreen quantitation, indicating contamination was not a problem. Amplicon pools were sequenced on an IlluminaHiSeq 2000 sequencer at the University of Colorado [62] . The stickleback diet-manipulation samples were sequenced on an IlluminaMiSeq to obtain paired-end 250 bp sequences. Data analysis was performed using QIIME [32] , [66] . Sequences were demultiplexed and quality filtered using default QIIME parameters (see Supplementary Note 1 for QIIME code). To focus the analysis on archaeal and bacterial taxa, 97% OTUs were picked using a closed-reference OTU picking protocol against the Greengenes database 12_10 release [67] prefiltered at 97% identity (available at http://greengenes.secondgenome.com/ ). Reads that did not match a reference sequence at >97% identity were discarded. The majority of discarded reads were either host mitochondrial 16S or had no BLAST match at all, and are probably sequencing error. Taxonomic assignments for OTUs were based on the Greengenes reference sequence defining that OTU and the Greengenes tree were used for computing phylogenetic diversity metrics. Lacking specific information about the function (or lack thereof) of the thousands of observed microbial OTUs, we analyse all observed OTUs (except photosynthetic cyanobacteria, <10% of total, which we removed). Some OTUs may not be long-term or functional natives of the hosts’ gut microbial community. We rarefied the data to 3,000 sequences per sample to calculate unweighted UniFrac [68] distances between samples, to obtain unweighted PCoA. As some statistics require rarefaction to equal coverage (for example, PCoA scores), we excluded individuals with fewer than 3,000 sequence reads from all analyses (starting with N =175 stickleback, 180 perch). Thus, sample sizes for analyses of PCoA data are slightly lower than sample sizes for GLM analyses that can retain all individual hosts, because they account for variable sequencing depth. Similar methods were used to identify mouse microbiota, as previously described [2] , [49] . The V4 region of the 16S rRNA gene was amplified using bar-coded fusion primers (F515/R806) with the 454 A Titanium sequencing adapter at the EnGenCore Facility at the University of South Carolina. The raw data from the 454 pyrosequencing machine were first processed through a quality filter that removed sequence reads that did not meet the quality criteria. Sequences were removed if they were shorter than 200 nucleotides, longer than 1,000 nucleotides, contained primer mismatches, ambiguous bases, uncorrectable barcodes, or homopolymer runs in excess of six bases. The remaining sequences were analysed using QIIME as described above. Data analysis Except where noted, the following analyses were conducted in R (ref. 69 ). Details of sequencing depth, microbial taxon composition and diversity, and frequencies and prevalences are given in Supplementary Data 1 . For each microbial taxonomic rank (phyla, class, order, family, genus and species), we determined the relative abundance of each taxon identified by Greengenes, out of all identified sequence reads for each individual (not rarefied). Within each host species, a large number of OTUs are found in only a single host individual. In wild-caught stickleback, 3,731 out of 8,880 OTUs (excluding cyanobacteria) are restricted to a single individual (3,731/9,290 for perch, 1,962/3,867 for lab-reared stickleback). These are not used in further analyses, as they contribute little to the leading PCoA axes and are not examined in GLM analyses of abundant OTUs. To compare microbial taxon relative abundance between host species or between sexes, we used Spearman rank correlations of taxon log relative abundance. To evaluate whether hosts or sexes differed in microbial OTU composition, we used multinomial GLMs testing whether microbial relative abundance depended on sex or species, with individual host as the level of replication. The multinomial GLM accounts for different sequencing depth for each host individual and hence does not require rarefying all individuals to the lowest common sequencing depth. As microbial communities may be spatially structured within the gut [70] , this difference in sampling method between host species (inevitable given their different sizes) may mean that some differences in gut microbiota between hosts is a consequence of sampling method (intestinal tissue sampled) rather than a difference between the two species. We used MANOVA analyses to test whether overall microbial community covaries with diet (α and tpos ), species, sex and all interactions. The dependent data in these MANOVAs are a matrix of individuals’ microbial PCoA scores, using axes collectively explaining 50% of the cumulative variation in microbial composition (PCoA1–27). MANOVAs are effective at detecting effects of individual explanatory variables on a dependent matrix, but are less effective at finding multivariate combinations of continuous predictor variables that jointly affect combinations of axes in a dependent matrix. For this purpose, we carried out CCA to identify multivariate axes of fish traits (diet and morphology) most strongly correlated with multivariate combinations of PCoA measures of the microbiota. CCA was first run for each species. As CCAs do not incorporate interactions with categorical factors (sex), we re-ran CCAs separately for each sex within each species. P -values for correlated axes were obtained by asymptotic approximations as implemented in the R package CCP. If CCAs identified the same axes of covariation in males versus females, then the loadings of the original traits on the CCA x and y axes should be similar (correlated) in males and females; thus, we tested for between-sex correlations in axis loadings. We tested whether host diet, species and sex influence the relative abundance of individual microbial taxa. Within each host species, we identified the most abundant OTUs with >0.01% mean relative abundance ( N =566 OTUs). Each abundant OTU was examined using a GLM with quasibinomial error to test whether the abundance of the OTU (number of sequences for the OTU, out of each individual hosts’ sequence read depth) depended on the hosts’ species, sex, diet (α and tpos ) and all interaction terms. Host diets were standardized to standard normal distributions to be comparable between species. GLMs are well suited for testing whether non-normally distributed response variables depend on continuous and/or categorical predictors and their interactions. In binomial GLMs, the response variable is a two-column matrix recording the number of times a given response was observed or not, thereby allowing us to account for sequencing depth of each host microbiota in our analyses without requiring loss of data through Rarefaction. Due to overdispersion seen in counts of microbial OTUs, instead of binomial GLMs, we use quasibinomial error that is less sensitive to outliers. To account for false positives (type I error) arising from multiple statistical comparisons we applied an FDR analysis to calculate q -values for each test. We also calculated the percentage of OTUs that exhibited significant GLM effects (at P <0.05) and used a Fisher’s exact test to evaluate whether this percentage exceeds the 5% null expectation. Note that when we do find an excess of significant diet effects (above 5% false positive rates), one does not necessarily know which particular microbial OTUs exhibit real diet effects, only that there is an excess of significant results indicating that some of the positive results are real. However, our primary goal is to demonstrate that sex*diet interactions affect microbial abundances in general; the goal of identifying the specific OTUs is secondary here. Applying these tests to only the OTUs with >0.05% or >0.1% mean relative abundance ( N =194 and 109 OTUs, respectively) yielded a higher fraction of significant results; thus, the results we report here are comparatively conservative. To interpret interactions between sex and diet, we repeated the GLMs to test for diet effects on each OTU, this time within each sex and species, and retained diet effect sizes in the form of estimated slopes (change in logit relative abundance per unit of the diet metric) divided by the s.e. of the slope. To test whether sexes exhibit similar diet effects on OTUs, we calculated Spearman rank correlations between diet effect sizes on OTUs in males, versus diet effects on the same OTUs in females. We use a similar approach to test for similarity in diet effects between host species (perch versus stickleback) and between lab versus wild stickleback. To determine whether males or females exhibit stronger microbial responses to diet (ignoring effect direction), we used Wilcoxon signed-rank tests to compare the males’ versus females’ absolute value of diet effects estimated from GLMs. We applied the preceding statistical approaches (MANOVA for multivariate measures of microbiota, GLMs for individual microbes) to test for sex*diet effects on PCoA scores and OTU relative abundances in the following: i Lab-reared stickleback fed littoral versus pelagic prey. Analysing the first experiment (males only), we also tested for a fixed effect of diet and a random effect of tank. Analysing the second experiment (both sexes), we tested for sex*diet interactions but no tank effect, because all fish were on a shared recirculating water supply. For each experiment, we used linear DFA to define combinations of PCoA axes that best distinguish treatment groups (and sexes in experiment two), and regressed each OTU on each DFA axis to identify microbes generating diet and sex*diet effects. ii Captive mice. As 454 sequencing provided lower sequence depth per individual, we had less resolution to infer OTU relative abundances, so we focus on genera. The MANOVA and GLMs included a random effect of mouse strain. iii Previously published human microbiota and diet data [15] . To obtain a manageable number of axes of diet variation in humans, we used principal component analysis of diet composition to score individuals along major axes of diet variation ( Supplementary Data 3 ), retaining the top nine principal component (PC) axes whose eigenvalues exceeded broken-stick null expectations. We used GLMs to test each abundant OTU (>0.1% mean relative abundance, N =125 OTUs) for sex, diet and sex*diet effects using each of the nine principal component (PC) axes separately. To account for multiple comparisons, we determined whether the number of OTUs with significant sex*diet interactions ( P <0.05) exceeded 5% null expectations attributable to statistical false positives. iv We used a similar GLM-based approach to test for sex*diet effects on the relative abundances of gene functional groups, inferred from PICRUSt [40] , a computational approach to predict the functional composition of a metagenome using marker gene data (for example, 16S rRNA amplicons) and a database of reference genomes as described in ref. 40 . Accession codes: Microbial sequence data and host metadata have been deposited in the European Nucleotide Archive (ENA), European Bioinformatics Institute, with accession codes ERP006029 , ERP006030 , and ERP006032 . How to cite this article: Bolnick, D. I. et al. Individual diet has sex-dependent effects on vertebrate gut microbiota. Nat. Commun. 5:4500 doi: 10.1038/ncomms5500 (2014).